Switching of myosin-V motion between the lever-arm swing and Brownian search-and-catch Motor proteins are force-generating nanomachines that are highly adaptable to their ever-changing biological environments and have a high energy conversion efficiency. Here we constructed an imaging system that uses optical tweezers and a DNA handle to visualize elementary mechanical processes of a nanomachine under load. We apply our system to myosin-V, a well-known motor protein that takes 72 nm 'hand-over-hand' steps composed of a 'lever-arm swing' and a 'Brownian search-and-catch'. We find that the lever-arm swing generates a large proportion of the force at low load (<0.5 pN), resulting in 3 k B T of work. At high load (1.9 pN), however, the contribution of the Brownian search-and-catch increases to dominate, reaching 13 k B T of work. We believe the ability to switch between these two force-generation modes facilitates myosin-V function at high efficiency while operating in a dynamic intracellular environment. Myosin-V is a dimeric motor protein that transports various cargos such as melanosomes, endoplasmic reticulum and messenger RNAs [1] , [2] by moving processively along cytoskeletal actin filaments [3] , [4] , [5] . Because of the cell's dense and heterogeneous actin meshwork [6] , the cargo itself should apply a dynamic load onto the myosin-V. To overcome this, a single myosin-V converts the chemical free energy of 1 ATP into a directional motion of 36 nm and a maximum force of 2–3 pN (refs 4 , 7 , 8 ). The energy conversion efficiency depends on external load, but can reach ~100% during a forward step near stall force [9] . The minimal unit for myosin-V force generation is a motor or head domain, which includes the actin and nucleotide-binding site, and a lever-arm, which has six calmodulin-binding motifs [10] , [11] . A crystal structure and electron micrographs have suggested the lever-arm tilts in conjunction with ATP hydrolysis cycle [12] , [13] , leading to the model assumes that the 'lever-arm swing' is the dominant process for force generation [14] , [15] . However, recent single-molecule nano-imaging and high-speed atomic force microscopy (AFM) have revealed that the two head domains alternately step 72 nm (hand-over-hand mechanism) [16] , [17] , [18] by combining the lever-arm swing [19] by the lead head with a 'diffusional Brownian search' by the rear head [17] , [20] . In general, the lever-arm swing is responsible for force generation and triggering the Brownian search following detachment of the rear head. We have argued, however, that the hand-over-hand mechanism in processive myosins also entails a Brownian search-and-forward-catch component, where attachment of the detached head to actin to the forward and backward binding sites is enhanced and suppressed, respectively, in a strain-dependent manner [21] , [22] and/or by a steric effect between the myosin head and sites [23] , [24] , a theory consistent with the A.F. Huxley Brownian ratchet model for muscle contraction [25] . To confirm whether the stroke or Brownian search is the greater contributor to force generation, we therefore sought to measure their energetic contribution. Here we describe a labelling method and measurement system of high spatio-temporal resolution that uses DNA as a nanometric tool [26] , finding that the contribution of the two mechanisms depends on the load. At low load (<0.5 pN), the lever-arm swing is dominantly responsible for force generation, contributing 3 k B T of work. At high load (1.9 pN), however, the contribution of the Brownian search-and-catch increases to dominate, reaching 13 k B T of work, whereas that from the lever-arm changes very little. We believe this switching mechanism is an important feature that allows myosin-V to adapt to a cell's dynamic environment. 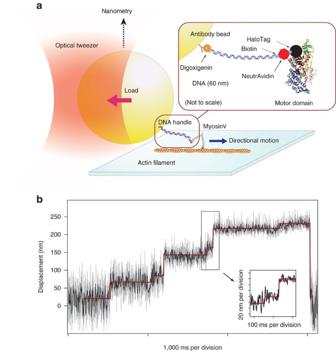Figure 1: Detection of the lever-arm swing and Brownian search-and-catch by a single myosin-V dimer. (a) Optical trap assay. Inset: illustration of the DNA-handle linking the myosin head and bead. The structure of the myosin head is obtained by modifying the figure from ref.27. (b) Processive steps of single myosin-V molecules at low ATP concentrations (3 μM). Consecutive 20+57 nm sub-steps movements are seen. Grey trace, data low-pass filtered at 400 Hz. Individual steps (red line) were detected by a runningt-test (Methods). Black trace, data median-filtered. Inset: sub-steps low-pass filtered at 200 Hz and enlarged. The trace was corrected by an attenuation factor (Methods). Lever-arm swing and Brownian search-and-catch under load Figure 1a shows our measurement system. One end of a double-stranded DNA (DNA handle, ~60 nm in length) was biotinylated and attached to the amino terminus of a myosin-V head via neutravidin. The opposite end was labelled with digoxigenin (DIG) and attached to a 200-nm fluorescent polystyrene bead coated with DIG antibodies. The bead was optically trapped and the position was detected with nanometric and millisecond spatio-temporal resolution. To prevent steric hindrance from the bead, the length of the DNA-handle was designed to be longer than the size of the myosin-V dimer (30–40 nm). Figure 1: Detection of the lever-arm swing and Brownian search-and-catch by a single myosin-V dimer. ( a ) Optical trap assay. Inset: illustration of the DNA-handle linking the myosin head and bead. The structure of the myosin head is obtained by modifying the figure from ref. 27 . ( b ) Processive steps of single myosin-V molecules at low ATP concentrations (3 μM). Consecutive 20+57 nm sub-steps movements are seen. Grey trace, data low-pass filtered at 400 Hz. Individual steps (red line) were detected by a running t -test (Methods). Black trace, data median-filtered. Inset: sub-steps low-pass filtered at 200 Hz and enlarged. The trace was corrected by an attenuation factor (Methods). Full size image Using this system at low ATP concentrations (3 μM) and low sampling rate (12.8 Hz), myosin-V was seen to take 77 nm processive steps ( Supplementary Fig. S1 ). The distribution of the dwell times between adjacent steps obeyed successive two rate-limiting reactions ( k =2.4 s −1 ), consistent with an ATP-binding rate of k =2.1–2.7 s −1 (refs 28 , 29 ) and second-order rate constants for ATP binding to acto-myosin-V of 0.7–0.9 μM −1 s −1 (refs 28 , 29 ).These results strongly suggest myosin-V linked to the optically trapped bead via the DNA handle and walked in a hand-over-hand fashion [16] . When the time resolution was improved to ~2 ms (Methods), we were able to observe 20 nm sub-steps ( Figs 1b and 2a ). Steps were resolved by computer-aided analysis based on a running t -test (Methods). Because the duration of the sub-steps was 123 ms, which is comparable to the first-passage time for a Brownian head to reach a forward actin-binding site 77 nm away under load ( Supplementary Fig. S2a–c ), and the expected bead displacement from the lever-arm swing is 20 nm (refs 30 , 31 , 32 , 33 ), we concluded the 77 nm steps to be composed of a 20-nm lever-arm swing and 57 nm Brownian search sub-step. Using 60-nm gold nanoparticles and no load, Dunn et al . reported the Brownian search to be 17 ms (ref. 17 ), a magnitude less than our result. Differences in the experimental designs likely explain this discrepancy, as the drag coefficient for our beads was 3.3-fold (200 nm/60 nm in diameter) larger than theirs, while the load applied slowed the diffusion time of the Brownian head exponentially [34] . We rule out the possibility of artificial steps caused by detachment of the rear head because the displacement expected by detachment of the rear head is negligible ( Supplementary Fig. S3 ). 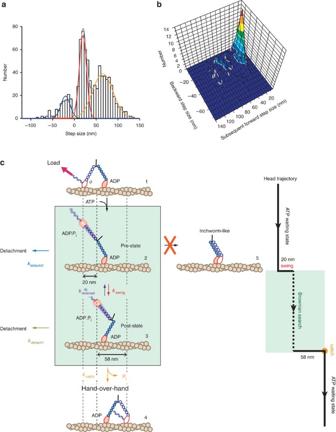Figure 2: Step size and scheme for myosin-V motion. (a) Distribution of step sizes at 3 μM ATP concentrations (N=796). The peak positions of a three Gaussian function fit were −20±11 nm (blue line), 20±8 nm (red line) and 65±24 nm (orange line) (mean±s.d.). (b) Correlation of step size for backward steps and the subsequent forward step size. The size of the backward step was plotted against the size of the subsequent step, creating a three-dimensional histogram of the data set (N=168). Most backward steps couple with 20 nm forward steps. This strong correlation suggests that ~40 nm inchworm-like steps (see (c)) are negligible. (c) Schematic diagram for myosin-V motility under load. The rear head binds ATP and detaches from actin (state 1→2 transition). A 20 nm sub-step results from a lever-arm swing (state 2→3 transition). The free head undergoes a Brownian search-and-catch to bind to the next actin-binding site, resulting in a 57-nm sub-step (state 3→4 transition). For the −20 nm peak, the lever-arm reverses its motion (state 3→2 transition). Detachment occurs only during the one-headed bound state (states 2 or 3). Inchworm-like steps are negligible (state 2→5 transition). The right schematic shows a head trajectory that traces a single motor domain during one ATP cycle. Figure 2: Step size and scheme for myosin-V motion. ( a ) Distribution of step sizes at 3 μM ATP concentrations ( N =796). The peak positions of a three Gaussian function fit were −20±11 nm (blue line), 20±8 nm (red line) and 65±24 nm (orange line) (mean±s.d.). ( b ) Correlation of step size for backward steps and the subsequent forward step size. The size of the backward step was plotted against the size of the subsequent step, creating a three-dimensional histogram of the data set ( N =168). Most backward steps couple with 20 nm forward steps. This strong correlation suggests that ~40 nm inchworm-like steps (see ( c )) are negligible. ( c ) Schematic diagram for myosin-V motility under load. The rear head binds ATP and detaches from actin (state 1→2 transition). A 20 nm sub-step results from a lever-arm swing (state 2→3 transition). The free head undergoes a Brownian search-and-catch to bind to the next actin-binding site, resulting in a 57-nm sub-step (state 3→4 transition). For the −20 nm peak, the lever-arm reverses its motion (state 3→2 transition). Detachment occurs only during the one-headed bound state (states 2 or 3). Inchworm-like steps are negligible (state 2→5 transition). The right schematic shows a head trajectory that traces a single motor domain during one ATP cycle. Full size image A second peak at 65 nm in the step size histogram ( Fig. 2a ) can be explained by convolving the 57 nm Brownian-search and 77 nm step when the 20 nm lever-arm swing could not be resolved (see Supplementary Discussion ). The third peak at −20 nm is probably due to lever-arm reversals (back steps), as these were seen to mostly couple with subsequent 20 nm lever-arm swings ( Fig. 2b ) [33] . Furthermore, correlating −20 nm steps with subsequent 20 nm steps suggests that inchworm-like steps, which have been observed in myosin-VI (ref. 35 ), were negligible ( Fig. 2b ). Schematically, inchworm-like steps would occur from the state 2→5 transition seen in Fig. 2c . Because the inchworm-like mechanism requires two ATP for every 72 nm step of a head (36 nm displacement of a tail), whereas the hand-over-hand mechanism only requires one ( Supplementary Fig. S4 ), we suggest myosin-V is designed to be an energy-efficient motor. ATP dependency of the stability in the lead head In the case of physiologically saturating ATP concentrations (1 mM), the −20-nm lever-arm swing reversal was more frequently observed ( Fig. 3a,b ). That we observed fewer backward steps at low ATP concentrations could be because the post-lever-arm swing conformation is more stable in the nucleotide-free state than in the ADP-bound state [18] , [33] , [36] , which increases with rising ATP concentrations, therefore reducing the likelihood of lever-arm swing reversals. 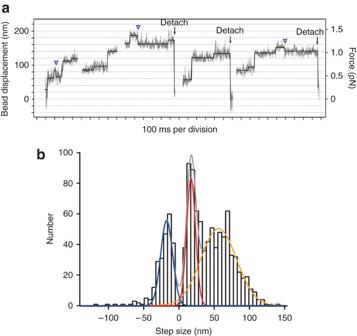Figure 3: Detection of 20 nm and −20 nm lever-arm swings. (a) Myosin motility at saturating ATP concentrations (1 mM). Grey traces, data low-pass filtered at 400 Hz. Individual steps (black line) were detected by a runningt-test (Methods). Blue arrowheads indicate −20 nm lever-arm reversals; black arrows indicate detachment events. (b) Distributions of step sizes at 1 mM ATP concentrations. Peak positions of a three Gaussian function fit show steps at −17±8 nm (blue line), 20±6 nm (red line), and 56±25 nm (orange line) (mean±s.d.).N=1,056. Figure 3: Detection of 20 nm and −20 nm lever-arm swings. ( a ) Myosin motility at saturating ATP concentrations (1 mM). Grey traces, data low-pass filtered at 400 Hz. Individual steps (black line) were detected by a running t -test (Methods). Blue arrowheads indicate −20 nm lever-arm reversals; black arrows indicate detachment events. ( b ) Distributions of step sizes at 1 mM ATP concentrations. Peak positions of a three Gaussian function fit show steps at −17±8 nm (blue line), 20±6 nm (red line), and 56±25 nm (orange line) (mean±s.d.). N =1,056. Full size image To estimate the probability of a nucleotide-free or ADP-bound state in the lead head, we calculated the dissociation rate of both heads. According to Oguchi et al . [37] , ADP dissociations from the lead and rear heads are given by respectively, where k ADP − is the rate of ADP dissociation; F , force; and k B T , thermal energy. Assuming the internal load is 1.5 pN when the lead head is in the pre-powerstroke state [33] , the ADP dissociation rate from the lead head is 1.3 s −1 , which corresponds to a time constant of 743 ms, and from the rear head is 21 s −1 , which corresponds to a time constant of 49 ms. At 3 μM ATP and 1 mM ATP, the dwell time of the rigour state for the rear head is 417 ms and only a few milliseconds, respectively [28] . Therefore, at low ATP concentration (3 μM), the time before ADP dissociation from the lead head (743 ms) is comparable to the time before ATP binding to the rear head (417+49=466 ms). On the other hand, at physiological ATP concentration (1 mM), the total dwell time of the rear head is only about 50 ms, which suggests that for much of the stepping time the lead head is in the ADP bound state. Thus, the population of the ADP bound state for the lead head increases with ATP concentration. Load-dependent kinetics of the lever-arm swing and reversal The durations of state 3 and 2 in Fig. 2c , τ 1 and τ 2 , respectively, were load-dependent ( Fig. 4a ) and fit to a single exponential curve. The inverse of the durations describes the transition rates (1/ τ 1 = k total1 = k reversal + k catch + k detach1 and 1/ τ 2 = k total2 = k swing + k inchworm-like + k detach2 ). The both durations ( τ 1 and τ 2 ) are affected not only by k reversal or k swing . Especially, τ 1 increase at higher load because k catch rapidly decreases depending on load. The ratios of the rates correspond to the frequency of the observed events ( k reversal : k catch : k detach1 = N reversal : N catch : N detach1 and k swing : k inchworm-like : k detach2 = N swing : N inchworm-like : N detach2 ; where N i is the number of observations for state i). In general, the above relationships include the rate constant for 40 nm forward inchworm-like steps. However, because these were negligible ( Fig. 2b,c ), we can assume k inchworm-like =0, simplifying the above relationships. 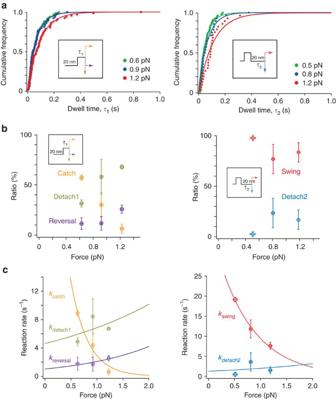Figure 4: Dwell time and frequency of the 20 nm and −20 nm lever-arm swings. (a) Cumulative frequency of dwell times for post- (left) and pre- (right) lever-arm swing states at different loads, respectively. The inverse of the durations equals the sum of each transition rate for each state (1/τ1=ktotal1=kreversal+kcatch+kdetach1and 1/τ2=ktotal2=kswing+kdetach2). Dwell times were fit to a single exponential function (seeMethodsand equation (1)) after removing data <60 ms. Inset: Schematic diagram of the transition pathways from the post- (left) and pre- (right) lever-arm swing states. Following a lever-arm swing, myosin-V takes one of the reversal, catch, or detach1 pathway. Assuming reversal, it next takes either the swing or detach2 pathway. (b) The normalized frequency of each transition state from the post- (left) and pre- (right) lever-arm swing states. The frequency of each transition was experimentally obtained by counting the number of reactions. Error bars show s.e.m. The frequencies were 67 at low load, 65 at middle load, and 66 at high load for the post-lever-arm swing state (left), and 27 at low load, 27 at middle load, and 28 at high load for the pre-lever-arm swing state (right). (c) Load dependencies of the reaction rateskcatch,kdetach1,kdetach2,kreversal, andkswingwere described by a single exponential (seeMethodsand equation (2)). Each plot was estimated by the load-dependency of the durations inFig. 4aand the frequency of each transition state inFig. 4b. Error bars show the s.e.m. Figure 4: Dwell time and frequency of the 20 nm and −20 nm lever-arm swings. ( a ) Cumulative frequency of dwell times for post- (left) and pre- (right) lever-arm swing states at different loads, respectively. The inverse of the durations equals the sum of each transition rate for each state (1/ τ 1 = k total1 = k reversal + k catch + k detach1 and 1/ τ 2 = k total2 = k swing + k detach2 ). Dwell times were fit to a single exponential function (see Methods and equation (1)) after removing data <60 ms. Inset: Schematic diagram of the transition pathways from the post- (left) and pre- (right) lever-arm swing states. Following a lever-arm swing, myosin-V takes one of the reversal, catch, or detach1 pathway. Assuming reversal, it next takes either the swing or detach2 pathway. ( b ) The normalized frequency of each transition state from the post- (left) and pre- (right) lever-arm swing states. The frequency of each transition was experimentally obtained by counting the number of reactions. Error bars show s.e.m. The frequencies were 67 at low load, 65 at middle load, and 66 at high load for the post-lever-arm swing state (left), and 27 at low load, 27 at middle load, and 28 at high load for the pre-lever-arm swing state (right). ( c ) Load dependencies of the reaction rates k catch , k detach1 , k detach2 , k reversal , and k swing were described by a single exponential (see Methods and equation (2)). Each plot was estimated by the load-dependency of the durations in Fig. 4a and the frequency of each transition state in Fig. 4b . Error bars show the s.e.m. Full size image Although we only observed 9 reversal events among the 68 events at low load ( Fig. 4b ), we cannot completely rule out a possibility that our experimental system poorly detects the lever-arm swing at low load, presumably due to the restricted time resolution or rotation of the bead. This means the step-size histogram may include unresolved 77 nm steps. If so, we cannot determine whether detachment occurs from the pre- or post-state at low load. This becomes a problem when analysing τ 2 , because the size of τ 2 depends on the state from which detachment occurs ( Fig. 4c ). Therefore, we exclude dwell times before detachment events for our analysis of τ 2 at low load, instead only analysing dwell times before lever-arm swings. Figure 4b shows the normalized frequencies of the subsequent transition state from states 2 and 3 used to estimate the transition rates in Table 1 and Fig. 4c . Table 1 Kinetic parameters obtained from the model analysis. 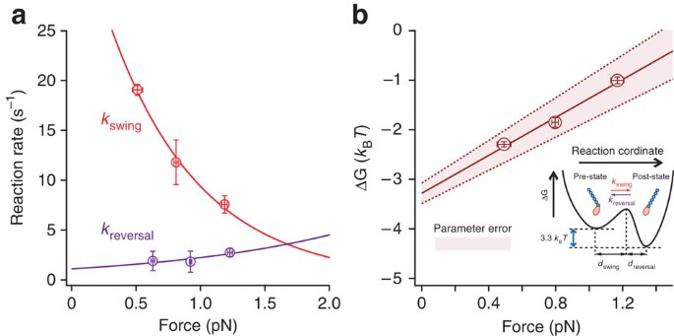Figure 5: Lever arm stability under load. (a) Reaction rates,kreversalandkswingplotted versus load. The load dependency can be described as a single exponential (seeMethodsand equation (2)). The characteristic distances,dreversalanddswing, are −2.9 nm and 5.9 nm, respectively (Table 1), meaning the energy barrier between the two states is asymmetrical. Thus, the lever-arm reversal is more robust to load than the lever-arm swing. The intersection of the two lines (1.7 pN) indicates the force at which pre- and post-lever-arm swing conformations occur at equal probability. The number of replicates studied is 26 at low load, 19 at middle load, and 15 at high loadfor kswing, and 9 at low load, 6 at middle load, and 17 at high load forkreversal. (b) Load dependency of the energy difference between the pre- and post-lever-arm swing states. Log(kreversal/kswing) is plotted versus load (seeMethodsand equation (4)). Each plot was estimated using plot data fromFig. 5a. ΔG was estimated to be −3.3kBTat no load. This value defines the maximum energy contribution of the lever-arm swing. Error bars show the standard error of the mean. Inset: Energy landscape of the two state lever-arm model. Full size table Figure 5a shows the load dependent transition rate for the lever-arm swing and the lever-arm reversal. The lever-arm swing involves a structural change that is opposed by the load. Therefore, the reaction rate decreases with increasing load in a manner that obeys an Arrhenius-type transition (Methods; equation (2)). In contrast, load should promote lever-arm reversal, which is consistent with our observation that the rate slightly increases with increasing load. The fitting parameter, d , which relates to the force dependency of the reaction, indicates the lever-arm reversal is less sensitive to load than the lever-arm swing ( Table 1 ). Therefore, once the lever-arm has swung, it robustly maintains the post-lever-arm swing conformation when sensing load. Figure 5: Lever arm stability under load. ( a ) Reaction rates, k reversal and k swing plotted versus load. The load dependency can be described as a single exponential (see Methods and equation (2)). The characteristic distances, d reversal and d swing , are −2.9 nm and 5.9 nm, respectively ( Table 1 ), meaning the energy barrier between the two states is asymmetrical. Thus, the lever-arm reversal is more robust to load than the lever-arm swing. The intersection of the two lines (1.7 pN) indicates the force at which pre- and post-lever-arm swing conformations occur at equal probability. The number of replicates studied is 26 at low load, 19 at middle load, and 15 at high load for k swing , and 9 at low load, 6 at middle load, and 17 at high load for k reversal . ( b ) Load dependency of the energy difference between the pre- and post-lever-arm swing states. Log( k reversal / k swing ) is plotted versus load (see Methods and equation (4)). Each plot was estimated using plot data from Fig. 5a . ΔG was estimated to be −3.3 k B T at no load. This value defines the maximum energy contribution of the lever-arm swing. Error bars show the standard error of the mean. Inset: Energy landscape of the two state lever-arm model. Full size image Distance parameter of the lever-arm swing The distance parameter for the swing ( d swing ) plus the distance parameter for the reversal swing ( d reversal ) should equal the total swing distance. However, because the bead displacement by the swing peaks at 13±5 nm (mean±s.d.) in the histogram without correction (data not shown), experimentally the total distance parameter d swing + d reversal should actually equal this displacement 13±5 nm, not 20 nm. Our finding that d swing + d reversal =8.8±1.7 nm ( Supplementary Table S1 ) is in agreement with the experimental 13±5 nm value. Free energy difference between the pre-and post-states Given the individual rate constants, we can estimate the free-energy difference (Δ G ) between the pre- and post-lever-arm swing states of the lead head by using the formula k reversal / k swing =exp((Δ G − F Δ x ) /k B T ), where F , Δ x , k B and T denote force exerted by the optical trap, the characteristic distance, Boltzmann's constant and absolute temperature (297±1 K), respectively ( Fig. 5b ). An electron microscopy study has found that 93% of lead heads are in the pre-lever-arm swing state when both myosin heads are bound to actin [36] . This corresponds to a Δ G= − k B T ln(0.07/0.93)=+2.5 k B T , which when extrapolating from Fig. 5b results in a 3.0-pN load (2.6–3.6 pN with a parameter error). This value agrees with other reports that found the intramolecular load in the two-headed bound state to be 1.5–3.5 pN (refs 33 , 37 ). At no load, which describes the maximum energy bias of the lever-arm swing, Δ G was estimated to be −3.3 k B T ( Supplementary Table S1 ). Because the ATP concentration was saturating, myosin-V should be predominantly in the ADP-bound state. In a conventional optical tweezers assay [4] , [7] , [8] , where myosin-V is loaded via the tail domain ( Fig. 6a , inset), myosin-V produces 18 k B T (2 pN×36 nm=72 pNnm) of work near stall force (2–3 pN). The work by a single lever-arm swing apparently seems to reach 10 k B T (2 pN×20 nm lever-arm swing), which is inconsistent with our estimate of the bias energy (3.3 k B T ). The discrepancy is reconciled in the discussion. 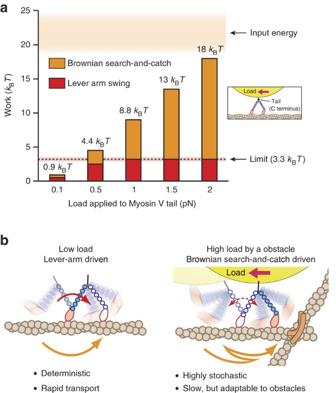Figure 6: Switching the mode of force generation. (a) Work done by myosin-V depends on the load applied to the tail (inset). Whereas the work done by the Brownian search-and-catch increases with load, that done by the lever-arm is constrained by the energy difference between the pre- and post-lever-arm swing states. (b) Model for myosin-V force generation. At low load, the contribution of the lever-arm swing to myosin-V movement is greater, making it a deterministic and rapid transporter. At high load, the contribution of the Brownian search-and-catch is greater, making myosin-V a stochastic and adaptable transporter. Figure 6: Switching the mode of force generation. ( a ) Work done by myosin-V depends on the load applied to the tail (inset). Whereas the work done by the Brownian search-and-catch increases with load, that done by the lever-arm is constrained by the energy difference between the pre- and post-lever-arm swing states. ( b ) Model for myosin-V force generation. At low load, the contribution of the lever-arm swing to myosin-V movement is greater, making it a deterministic and rapid transporter. At high load, the contribution of the Brownian search-and-catch is greater, making myosin-V a stochastic and adaptable transporter. Full size image Maximum work done by the Brownian search-and-catch The work done by a myosin dimer can be divided into two parts, work done by structural changes in the lever-arm and work done by the Brownian search-and-catch [17] , [20] . We showed hand-over-hand stepping is triggered by a 3.3 k B T lever-arm swing in the lead head. The Brownian-search-and-forward-catch contributes work to this system as load is exerted onto the myosin molecule. During physiological vesicle transport, myosin-V apparently distributes the load from a cargo bound to the tail domain completely onto the lead head. However, when the rear head undergoes Brownian motion, the lever-arm in the lead head should bend 10–15 nm backwards when a 2–3 pN load is exerted (bending stiffness=~0.2 pN/nm (ref. 38 )). In these cases, the Brownian head will conduct work when it catches an actin target 72 nm forward. Therefore, estimation of how large work the Brownian search-and-catch can potentially generate has significant meaning. We found that the majority of myosin-V molecules completed the Brownian search-and-catch against 0.93 pN on average (data not shown). This equates to a Brownian search-and-catch contribution of 13 k B T (57 nm×0.9 pN) of work, which is similar to the energy released from the Pi release (12 k B T ) (ref. 34 ) ( Fig. 2c ). Here we analysed the lever-arm swing and Brownian search-and-forward-catch done by the lead and rear heads, respectively, during myosin-V hand-over-hand steps. Attaching a 200-nm bead and applying a load to one myosin head sufficiently slowed the stepping process, allowing us to estimate the energetic contributions of these two processes. Furthermore, we could observe lever-arm reversals during hand-over-hand steps, which could not be seen in previous nano-imaging studies that used fluorescent dyes [16] and gold nanoparticles [17] or high-speed AFM observations [18] , because these used unloaded conditions. Surprisingly, the reversal occurred under 1 pN load (less than half of stall force (2–3 pN as a dimer)) and the estimated free-energy difference between the pre- and post-lever-arm swing states was 3.3 k B T , which is much less than the total work near stall force (18 k B T ). Is the 3.3 k B T energy bias of lever-arm swing sufficient to produce 2–3 pN force and 18 k B T total work at high load? On the basis of our results, the rates for the pre- and post-lever-arm swing states are equal at 1.7 pN ( Fig. 5a ). However, using the load dependency of the energy difference between the pre- and post-lever-arm swing states described in Fig. 5b , we can show that when 2.5 pN force is applied to the tail, Δ G is +1.5 k B T . This translates into only 19% of the lead heads swinging forward or being in the post-lever-arm swing state ( Fig. 2c , state 2→3). However, because k catch is sufficiently fast, this 19% is almost assured of advancing to state 4 to complete the step ( Supplementary Fig. S5 ). Thus, while the lever-arm swing seems to generate >10 k B T of work (>2 pN ×20 nm lever-arm swing), the majority of this actually comes from the forward catch. In conventional optical trapping nanometry (tail loading), myosin-V showed ~±20 nm half-steps within 36 nm regular steps at near stall forces of 1.7–3.0 pN (refs 4 , 7 , 8 ). Our results show that the 20 nm forward and backward steps originate from lever-arm swings and reversals by the lead head during the one-headed bound state ( Fig. 2c , state 2–3). Using our measurement system (head loading), we could observe −20 nm lever-arm swing reversals at less than 1 pN, because the geometry of our system slowed the time for the Brownian head to catch forward. In a conventional tail-loading condition, the Brownian head diffuses relatively freely, and rapidly catches forward actin before lever-arm swing reversal occurs such that ~20 nm steps are only observed at high load (see arrows in Supplementary Fig. S5b ). Electron microscopy results have suggested that the lever-arm in the lead head is fully populated in the pre-lever-arm swing state (93%) because of an intramolecular load [36] that is consistent with our results. On the other hand, Sellers and Veigel reported that the probability between the lever arm-swing and reversal states in single heads are equal at ~4 pN load [33] . This difference is likely because their definition of the lever arm-swing and reversal rate is different from ours. Whereas they defined the lever arm-swing and reversal rate as the reciprocal of the average dwell time in the pre-state and post-state, respectively, we obtained the lever arm-swing and reversal rate by subtracting other rates such as the detachment and catch rate from the reciprocals of the average dwell times (see Results and Supplementary Discussion ). Additionally, the difference in the force application geometry may partially explain the discrepancy. Figure 6a shows the contribution of the lever-arm swing and Brownian search-and-forward-catch for total myosin-V work at various loads when assuming conventional nanometry (tail loading) or physiological vesicle transport geometry. When 0.5 pN force is applied to the tail end, the lever-arm swing conducts 2.4 k B T (20 nm×0.5 pN) of work, whereas the total work done by the myosin-V is 4.4 k B T (36 nm×0.5 pN), meaning the Brownian search-and-catch component is 2.0 k B T . Although the amount of work done by the lever-arm swing increases with load, it never exceeds 3.3 k B T at saturating ATP concentrations (ADP-bound state). Any residual work then done by the Brownian search-and-catch actually dominates at high loads. Thus, our results argue the myosin-V is a lever-arm-driven motor under low loads, but a Brownian search-and-catch driven motor under high ones ( Fig. 6b ). This suggests that myosin-V can change its force-generating mechanism depending on the external force applied to the tail. Knowing that the vast majority of work done by myosin-V at high load is a stochastic process (Brownian search-and-catch) and that the proportion of work done by the deterministic lever-arm swing and Brownian search-and-catch varies with load offers important insights into the mechanisms used by myosin-V for its function. The hand-over-hand steps caused by deterministic lever-arm swings would be advantageous for smooth rapid movement at near-zero load when no obstacles are present ( Supplementary Movie 1 ). However, cells contain a cytoskeleton meshwork and a number of dynamic molecules and vesicles that risk disturbing transport [39] . In these cases, the Brownian search-and-catch mechanism should be advantageous for avoiding such obstructions ( Supplementary Movie 2 ). Thus, our findings indicate that myosin-V is an optimized nanomachine that is highly adaptable to its intracellular environment. These results should have significant implications on the design of artificial nanomotors. That the Brownian search-and-catch significantly contributes to force generation in myosin-V challenges the theory that biological molecular motors, such as myosin, kinesin and dynein, generate force primarily from a structural change [14] , [15] , [40] , [41] (in the case of myosin-V, this is the lever-arm swing). More likely, the work distribution between the structural change and the Brownian search-and-catch would vary with the molecular motor. The Brownian search-and-catch would be favourable for myosin-V, because it robustly moves long distances (several micrometers) through a diverse cellular environment. Other long distant transporters like kinesin and dynein might have similar features. In fact, a previous report has estimated that the contribution of the structural change in kinesin-1, called neck linker docking, is ~1.2 k B T (ref. 42 ). On the other hand, muscle myosin (myosin-II) may depend more on the structural change component for force as the region that muscle myosin functions is more constrained. Myosin construct Human Myosin-V-HMM heavy chain construct: pFB1-flag-HT-hMyosinVaHMM-Myc. The 3′ end [bp 3714 to 5484] of the Human Myosin-Va complementary DNA (ORK07567) was deleted to obtain a Myosin-Va-HMM cDNA fragment (encoding a.a. Met 1 -Thr 1238 ). This fragment includes the motor, neck, and coiled-coil domains. Flag-tag and HaloTag (DHA, Promega) fragments were attached at the 5′ end of the myosin-Va cDNA fragment for purification and biotin labelling; Myc-tag was attached at the 3′ end for detection. The Flag-HT-hMyosin-VaHMM-Myc fragment was introduced into the Baculovirus expression vector pFastBac1 between the BamHI and HindIII sites. Human calmodulin construct: pFB-hCaM. The calmodulin coding sequence (Kazusa, ORK11793) was also inserted into pFastBac1 between the BamHI and HindIII sites. Protein expression and purification Recombinant viruses for myosin-V heavy chain and calmodulin were produced by homologous recombination using the Bac-to-Bac Baculovirus Expression System (Invitrogen). Sf9 insect cells were maintained in a monolayer culture in ventilated 175 cm 2 flasks at 28 °C with 10% FBS (Invitrogen) and 1×Antibiotic-Antimycotic liquid (Invitrogen) /EX-Cell 420 (SAFC Biosciences). After co-infection at an multiplicity of infection of 1 and 0.5, respectively, and incubation for 60 h, cells were collected by centrifugation at 6,000 g for 5 min and stored at −80 °C. Frozen cells were suspended and sonicated in 10 ml per g cells of Lysis solution (30 mM Tris–HCl pH 8.0, 200 mM NaCl, 1 mM EGTA, 5 mM MgCl 2 , 5 mM ATP, and 0.05 mM DTT) containing Complete EDTA-free (Roche Diagnostics). After ultra centrifugation at 10,000 g for 20 min, soluble fractions were mixed with pre-activated Flag-affinity resin (ANTI-FLAG M2 Affinity Gel, Sigma) for 1 h. After removal of the unbound protein, 1 ml Lysis solution and 1.25 μl HaloTag PEG-Biotin Ligand (Promega) were added at a molecular ratio of 1:3 to the resin, which was lightly incubated on ice for 10 min to achieve N-terminal biotinylation. Afterward, Wash solution (30 mM Tris–HCl pH 8.0, 200 mM NaCl, 0.1 mM EGTA, 2 mM MgCl 2 , 2 mM ATP, and 0.05 mM DTT) was added to remove any unreacted reagent. Biotinylated protein was eluted by Elution solution (30 mM Tris–HCl pH 8.0, 200 mM NaCl, 0.1 mM EGTA, 2 mM MgCl 2 , 2 mM ATP, and 0.05 mM DTT) including 0.15 mM Flag peptide. The obtained myosin-V recombinant (~0.3 mg ml −1 ) was aliquoted and stored at −80 °C until use. Biotinylation was confirmed by using a streptavidin-alkaline phosphatase conjugate and bromochloroindolyl phosphate/nitro blue tetrazolium as the substrate. All steps were performed at less than 4 °C. Biotinylated and DIG-labelled DNA linker preparation A DNA linker (174 bp) was obtained from a pBluescript II KS(−) Plasmid using PCR amplification and a DNA fragment purification system (Wizard PCR Preps DNA Purification System, Promega). Primers for the PCR amplification were as follows. Biotinylated T7 primer, 5′ Biotin-CGCGTAATACGACTCACTATAG-3′; and DIG-T3 primer, 5′ AminoC6+Digoxigenin-GCGCAATTAACCCTCACTAAAG-3′. DNA-bead labelling A 174-base-pair double-stranded DNA oligomer was synthesized with digoxigenin at the 5′ end of one strand and biotin at the 5′ end of the other. A solution of double-stranded DNA oligomers was mixed at 1,000-hold molar excess with neutravidin. For all incubations and experiments, buffers contained 25 mM KCl, 20 mM HEPES-KOH (pH 7.8), 5 mM MgCl 2 and 1 mM EGTA. Carboxylate modified polystyrene beads (Invitrogen; 0.2 μm in diameter) were crosslinked to polyclonal anti-digoxigenin (Roche) and coated with 10 mg ml −1 BSA. The beads were incubated with a DNA solution that was previously mixed with neutravidin for 30 min at 4 °C. After incubation, the beads were linked to DNA via anti-DIG antibodies and centrifuged to remove excess neutravidin. Myosin-V was then mixed with the DNA-linked beads at an adjusted ratio such that 30% of the beads displayed movement. Single-molecule assay Fluorescently labelled actin filaments were quickly flowed into sample chambers in which α-actinin was directly adhered to a glass slide. The glass surface was then coated with 5 mg ml −1 casein. Single-molecule assays were performed at 24±1 °C in buffer containing 0.05% tween, ATP (1 mM or 3 μM) and ATP regenerase (0.1 mg ml −1 creatine kinase and 2 mM creatine phosphate) and an oxygen scavenger system (0.11 mg ml −1 glucose oxidase, 18 μg ml −1 catalase, 2.3 mg ml −1 glucose and 0.5% 2-mercaptoethanol). Instrumentation and data analysis Myosin-V tagged to a bead via the DNA-handle was optically trapped and brought to single actin filaments on the cover glass by observing its fluorescent image. Nanometry of the optically trapped bead was done by projecting the dark-field image onto a quadrant-photodetector with a response time of ~50 μs (ref. 22 ). Data were sampled at 24 kHz with a bandwidth of 10 kHz. Step sizes and dwell times of sub-steps were analysed automatically by a custom software (LABVIEW 9.0) or by eye. There was no significant difference between the two methods. Data were 400 Hz low-pass filtered before step detection. t -test values were calculated from low-pass filtered time series of the mean displacement and variance using a running time window of five data points. To determine step sizes, we calculated the time-averaged displacement between preceding step changes. Amplitudes were calculated relative to the preceding step. Bead displacement was corrected by an attenuation factor [43] such that step sizes include bending in the lever arm and stretching of the DNA-handle. The initial step of processive movement and its corresponding dwell time were not included in the analysis. Dwell-time distributions of pre- and post-states were plotted as cumulative and normalized distributions. The transition rate, k total , was obtained by least-squares fitting the model function: where t is time, F is force, P is probability, and i =1 or 2. Load dependency of the reaction rates was described by an Arrhenius-type transition: where k 0 is the transition rate in the absence of load, F is force, d is the characteristic distance, k B T is the thermal energy, and j =[swing, catch, detach1, detach2, or reversal]. Load dependency of the energy difference between the pre- and post-lever-arm swing states was also described by an Arrhenius-type transition: Taking the natural logarithm of equation (equation (3)) gives, How to cite this article: Fujita, K. et al . Switching of myosin-V motion between the lever-arm swing and Brownian search-and-catch. Nat. Commun. 3:956 doi: 10.1038/ncomms1934 (2012).